Selective ingress of a Samoan plume component into the northern Lau backarc basin Intra-plate basalt isotopic trends require mixing between enriched mantle components (EM1, EM2, HIMU) and a primordial component with high 3 He/ 4 He termed FOZO. However, proportions of components, geometric distributions within individual plumes, relative proportions of melting components and loci of mixing of melts and residues remain poorly understood. Here we present new Hf-Nd isotopic data of dredged sea floor basalts from the northern Lau backarc basin, ~250 km south of the subaerial and submerged Samoan chain, with high 3 He/ 4 He, 20 Ne/ 22 Ne and primordial 129 Xe/ 130 Xe, characteristic of the FOZO component. Combined Hf-Nd-noble gas isotope systematics require mixing of refractory, sub-northwestern Lau backarc mantle only with a spatially restricted FOZO component, most plausibly sourced from part of the Samoan plume. Other geographically restricted and possibly volumetrically minor enriched Samoan plume components are not detectable in northern Lau backarc samples, consistent with selective plume ingress of the FOZO component beneath the basin. Juxtaposition of the Samoan island chain north of the Tonga arc-Lau backarc basin provides a fortuitous opportunity, through geophysical and geochemical methods, to study the distribution in space and time of mantle flow patterns, both underlying the basin and to the north in the vicinity of Samoa. The largest, and still volcanically active Samoan islands of Savai’i and Upolu, are now along strike of the axis of the northernmost Tonga arc, separated from the latter by the WNW-trending Tonga Trench ( Fig. 1 ). On the basis of strongly elevated 3 He/ 4 He in the basin’s backarc magmas, southward ingress of the mantle plume tapped during formation of Samoa has been proposed [1] , [2] , [3] , [4] , [5] , [6] , [7] . There is convincing evidence the Samoan chain is formed from the partial melting of a mantle plume [8] , [9] , [10] , [11] , [12] . The Samoan islands are remarkable in that all of the five distinctive geochemical components that currently exist in the Earth’s mantle are manifest in the isotopic compositions of the Samoan lavas [13] . Extensive geochemical studies have revealed a spectrum of geochemically diverse mantle sources must be involved including the archetypal ‘enriched mantle 2’ (EM2) component with the highest 87 Sr/ 86 Sr (~0.720) yet discovered in ocean island basalt (OIB) [14] . Samoan magmatism samples a mixture of mantle sources that range from a ubiquitous low 87 Sr/ 86 Sr to high 3 He/ 4 He end-member component (Focal Zone–Austral (FOZO-A ref. 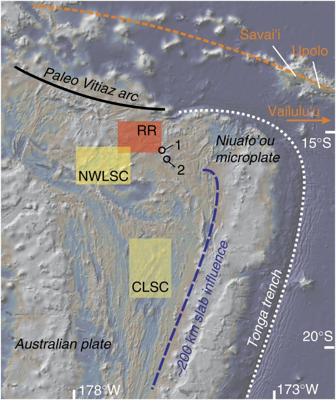Figure 1: Overview map of the greater study area. North of the Paleo-Vitiaz Trench is the presumed plume track (orange dashed line) for the Samoan Plume. The Rochambeau Rifts (RR) and parts of the Northwest Lau Spreading Centre (NWLSC) have geochemical signatures akin to oceanic island basalts43, whereas the Central Lau Spreading Centre (CLSC) has ultra-depleted mantle wedge geochemical signatures. A subduction overprint is not observed beyond ca 200 km west of the Tonga-Kermadec arc (blue dashed line). 1: submarine Dugong Volcano; 2: subaerial Niuafo’ou Island. The map is taken from the Global Multi-Resolution Topography (GMRT) synthesis60. 15 , 16 ) separately to EM2, but also to enriched mantle 1 (EM1), high-μ (high 238 U/ 204 Pb, HIMU) and a depleted mid-ocean ridge basalt (MORB) mantle (DMM; [13] see Table 1 for an overview of mantle components). Figure 1: Overview map of the greater study area. North of the Paleo-Vitiaz Trench is the presumed plume track (orange dashed line) for the Samoan Plume. The Rochambeau Rifts (RR) and parts of the Northwest Lau Spreading Centre (NWLSC) have geochemical signatures akin to oceanic island basalts [43] , whereas the Central Lau Spreading Centre (CLSC) has ultra-depleted mantle wedge geochemical signatures. A subduction overprint is not observed beyond ca 200 km west of the Tonga-Kermadec arc (blue dashed line). 1: submarine Dugong Volcano; 2: subaerial Niuafo’ou Island. The map is taken from the Global Multi-Resolution Topography (GMRT) synthesis [60] . Full size image Table 1 Overview of main mantle components. Full size table The Earth’s upper mantle, as sampled by MORBs, is depleted in incompatible elements consequent to the long-term sequestration of the latter in the continental crust [17] , outgassed in noble gases by melt extraction relative to primitive mantle, and at least locally, re-fertilized by whole-mantle advective processes [18] . On the other hand, some OIBs, including Samoa, have elevated 3 He/ 4 He and other distinct noble gas isotopic systematics compared with MORB [19] , [20] , [21] , requiring a distinctive source reservoir characterized either by relatively low U/He and/or lesser extents of outgassing [19] , [20] . Enriched mantle components (EM1, EM2, HIMU) prevalent in global OIB and characterized by distinctive radiogenic Sr-Pb-Nd-Hf isotope systematics [22] , [23] , [24] , [25] converge in multi-isotope space on the high 3 He/ 4 He FOZO component equivalent to the ‘primitive He mantle’ [8] or common (C) component [26] . Although the 3 He/ 4 He of MORB is ~8 × atmospheric, that of FOZO exceeds ~35 × atmospheric [21] . On the basis of distinction of FOZO and DMM, particularly in terms of noble gases, mantle plumes with OIB as their likely surface expression, have been postulated to originate in the deeper (relatively undegassed) mantle [19] . Geochemical mapping of OIB has revealed consistent spatial isotopic distributions in volcanic island chains, first observed for Hawaii [27] , [28] , and subsequently for the Samoan, Marquesas, Tristan-Gough and Society islands [13] , [29] , [30] , [31] , [32] . A bilateral conduit that inherits its isotope distribution from large-scale heterogeneity in the source of the mantle plume has been invoked to explain these characteristics. Current debate on plume structure is mostly focused on variations relating to distributions between enriched components, whereas the possible role of FOZO and modes of mixing between FOZO and enriched mantle components remains elusive. The remarkable isotopic variations of the Samoan chain [13] together with the potential for diversion of the Samoan mantle source(s) southwards into the opening Lau backarc basin permits some further exploration of spatial distribution of plume components. As the Tonga arc has rotated clockwise, because of an ultra-fast rollback of the subducting Pacific Plate, a number of spreading centres and rift zones have created the Lau Basin and led to the abandonment of the Lau Ridge as a remnant arc. Rapid rotation, resulting in a very high convergence rate with the Pacific Plate (~240 mm a −1 ), means meridional separation of the northern terminus of the Tonga arc with the primary Samoan hot-spot locus [12] (submarine volcano Vailulu’u [33] ) has progressively decreased. Toroidal flow of Pacific mantle around the foundering northern edge of the subducting Pacific Plate and into the widening Lau Basin has been proposed on the basis of He, Ne and Xe isotopic characteristics in the basin’s backarc magmas [1] , [2] , [4] , [7] , [34] and inferred arc-parallel seismic anisotropy by shear wave splitting related to olivine grain alignment in the mantle wedge [35] , [36] , [37] . A wide range of volcanic rock compositions has been discovered in the Lau Basin. These range from subduction-unaffected ridges and rifts in the northwest (Central Lau Spreading Centre (CLSC); Northwest Lau Spreading Centre (NWLSC); Rochambeau Rifts (RR), Fig. 1 ) to strongly subduction-overprinted spreading centres (Valu Fa Ridge and Fonualei Rifts) adjacent to the Tonga arc in the Southeast [5] , [38] , [39] , [40] , [41] , [42] , [43] , [44] . Superimposed on these geochemical features is the presence of two isotopically distinct mantle domains, identified primarily by Pb isotope compositions in dredged seafloor samples in the north-western and south-eastern Lau Basin, respectively [39] , [45] , [46] . Pacific-type mantle is dominant in the southern and western Lau Basin, and so-called Indian-type-mantle is predominant in the north-west. In this contribution, we present new high-precision Hf-Nd isotope data for exactly the same samples previously analysed for He and Ne isotopes [1] , [2] , and compare these with other published isotopic data for the Lau Basin and the Samoan chain. The combined isotopic data for the northwestern Lau Basin range from a local mantle wedge comprising a DMM source (Indian- or SOPITA-type [45] ) to values generally characteristic of FOZO, and not the EM1, EM2 or HIMU components manifest in surficial expressions of the Samoan Plume. We conclude selective ingress of some part of the Samoan Plume beneath the Lau Basin is occurring. Sampling and previous analyses Samples from this study were dredged during a research voyage (SS02/2009; NoLauVE) of Australia’s Marine National Facility, the RV Southern Surveyor [47] . Aliquots of the same glass samples from the RR, NWLSC, Dugong Volcano (DV) and the CLSC ( Fig. 1 ) have been previously analysed for major and trace element abundances [43] , He and Ne isotope compositions [1] , [2] . The DV is located ~100 km east of the southern end of the RR, 20 km northwest of the subaerial volcano of Niuafo’ou [42] , [48] . Separate glass samples from the same dredge hauls have been independently analysed for major and trace elements (including volatiles), Sr-Nd-Pb-Hf isotopes [41] and a subset of those for Xe isotopes [3] . 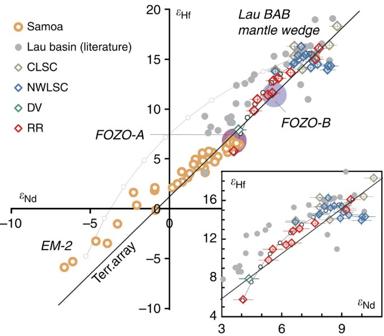Figure 2: Hf-Nd isotope co-variations in Northern Lau samples. A well-constrained mixing trend between local mantle wedge compositions (represented by Central Lau Spreading Centre (CLSC) samples61) and a Samoan Focal Zone Austral (FOZO-A) but not FOZO-B (Borealis) component is illustrated for the data presented here. Samples from the Northwest Lau Spreading Centre (NWLSC) and Dugong Volcano (DV) fall on this trend. Other samples from the Lau Basin (including illustrated literature data)41,45,54fall off this trend but may include older samples that are not related to the current plate tectonic setting, that is, may relate to the Vitiaz subduction zone, or some inter-laboratory inconsistency. Samples from the northernmost Lau Basin at the Rochambeau Rifts (RR) exhibit OIB-type isotope compositions that plot on a mixing trend with Samoan shield lavas55, which is isotopically identical to FOZO-A16. There is no apparent evidence for enriched mantle-2-type (EM2) signatures, that is, archetype for the Samoan plume. The mixing line between local depleted Lau mantle wedge is defined by: (176Hf/177Hf=0.28324,143Nd/144Nd=0.51313, Nd/Hf=5) and the Samoan FOZO-A mantle (176Hf/177Hf=0.282945,143Nd/144Nd=0.512838, Nd/Hf=13). The EM2 component is assumed to plot on the lower (that is, crustal) end of the Hf-Nf isotope array for Samoa55(176Hf/177Hf=0.28277,143Nd/144Nd=0.5125) Hf-Nd isotope compositions of Lau backarc basin samples The new Hf and Nd isotopic data are presented in Table 2 and shown in Fig. 2 . Isotopic data previously obtained in our laboratory using the same methods for the CLSC and tabled in Nebel et al . [49] are shown for comparison. Hafnium and Nd isotope compositions for the RR range from DMM-like ( ε Hf =+16.1 and ε Nd =+9.4) towards less radiogenic values, that is, ε Hf =+5.8 and ε Nd =+4.1, indicative of the involvement of time-integrated lower Lu/Hf–Sm/Nd mantle source component(s) than DMM. Samples from the NWLSC have a narrower spread from ε Hf =+16.3 to +13.8 and ε Nd =+10.2 to +6.7, respectively. The DV has ε Hf and ε Nd similar to the least radiogenic sample from the RR. In Fig. 3 , the 143 Nd/ 144 Nd versus 3 He/ 4 He, a plot previously used to identify primordial components [50] , determined on the same aliquots for our sample set from northwestern Lau Basin are shown for comparison; the available data from Samoa are also displayed [16] . Table 2 Hf-Nd isotope data for northern Lau backarc basin samples. Full size table Figure 2: Hf-Nd isotope co-variations in Northern Lau samples. A well-constrained mixing trend between local mantle wedge compositions (represented by Central Lau Spreading Centre (CLSC) samples [61] ) and a Samoan Focal Zone Austral (FOZO-A) but not FOZO-B (Borealis) component is illustrated for the data presented here. Samples from the Northwest Lau Spreading Centre (NWLSC) and Dugong Volcano (DV) fall on this trend. Other samples from the Lau Basin (including illustrated literature data) [41] , [45] , [54] fall off this trend but may include older samples that are not related to the current plate tectonic setting, that is, may relate to the Vitiaz subduction zone, or some inter-laboratory inconsistency. Samples from the northernmost Lau Basin at the Rochambeau Rifts (RR) exhibit OIB-type isotope compositions that plot on a mixing trend with Samoan shield lavas [55] , which is isotopically identical to FOZO-A [16] . There is no apparent evidence for enriched mantle-2-type (EM2) signatures, that is, archetype for the Samoan plume. The mixing line between local depleted Lau mantle wedge is defined by: ( 176 Hf/ 177 Hf=0.28324, 143 Nd/ 144 Nd=0.51313, Nd/Hf=5) and the Samoan FOZO-A mantle ( 176 Hf/ 177 Hf=0.282945, 143 Nd/ 144 Nd=0.512838, Nd/Hf=13). 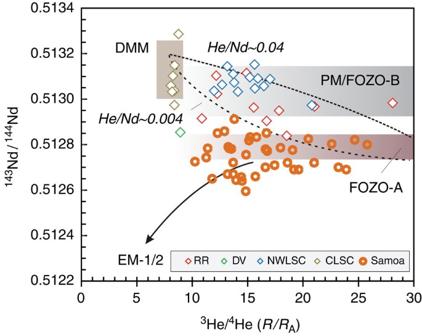Figure 3: Nd-He isotope composition of Lau Basin rocks in comparison to Samoan shield lavas. The grey field marks primitive mantle (PM) or Focal Zone Borealis (FOZO-B)62. Samoan samples63are characterized by a lower143Nd/144Nd, typified as Focal Zone Austral (FOZO-A)16. Mixing proportions between end-members are unconstrained because of unknown concentrations in those end-members, especially for He. End-member compositions estimated here are FOZO-Borealis (FOZO-B)50:143Nd/144Nd~0.5130, FOZO-A55:143Nd/144Nd~0.512838 as shown inFig. 2; both with [Nd]~13 p.p.m.,R/RA~35 with [He]~1 μg per c.c.m.; depleted MORB mantle (DMM)64:143Nd/144Nd~0.5132 with [Nd]~10 p.p.m.,R/RA~8 with [He]~0.5 μg per c.c.m.; representing the local mantle; EM214:143Nd/144Nd~0.5118 with [Nd]~27 p.p.m.,R/RA~0.05 with [He]~0.1 μg per c.c.m.; The two individual mixing lines represent different He/Nd (as indicated) with a 20 × lower He concentration of the lower mixing line in FOZO-A. CLSC, Central Lau Spreading Centre; DV, Dugong Volcano; NWLSC, Northwest Lau Spreading Centre; RR, Rochambeau Rifts; the arrow indicates a hypothetical mixing trend with enriched mantle components. The EM2 component is assumed to plot on the lower (that is, crustal) end of the Hf-Nf isotope array for Samoa [55] ( 176 Hf/ 177 Hf=0.28277, 143 Nd/ 144 Nd=0.5125) Full size image Figure 3: Nd-He isotope composition of Lau Basin rocks in comparison to Samoan shield lavas. The grey field marks primitive mantle (PM) or Focal Zone Borealis (FOZO-B) [62] . Samoan samples [63] are characterized by a lower 143 Nd/ 144 Nd, typified as Focal Zone Austral (FOZO-A) [16] . Mixing proportions between end-members are unconstrained because of unknown concentrations in those end-members, especially for He. End-member compositions estimated here are FOZO-Borealis (FOZO-B) [50] : 143 Nd/ 144 Nd~0.5130, FOZO-A [55] : 143 Nd/ 144 Nd~0.512838 as shown in Fig. 2 ; both with [Nd]~13 p.p.m., R/R A ~35 with [He]~1 μg per c.c.m. ; depleted MORB mantle (DMM) [64] : 143 Nd/ 144 Nd~0.5132 with [Nd]~10 p.p.m., R/R A ~8 with [He]~0.5 μg per c.c.m. ; representing the local mantle; EM2 [14] : 143 Nd/ 144 Nd~0.5118 with [Nd]~27 p.p.m., R/R A ~0.05 with [He]~0.1 μg per c.c.m. ; The two individual mixing lines represent different He/Nd (as indicated) with a 20 × lower He concentration of the lower mixing line in FOZO-A. CLSC, Central Lau Spreading Centre; DV, Dugong Volcano; NWLSC, Northwest Lau Spreading Centre; RR, Rochambeau Rifts; the arrow indicates a hypothetical mixing trend with enriched mantle components. Full size image To detect invasion of the Samoan Plume into the northern Lau Basin, the composition of the sub-Lau mantle free of ingress has to be determined. Geochemical studies [41] , [43] of latitudinal variations northwards from the CLSC through the NWLSC to the RR have demonstrated significant compositional changes. It should be noted that none of these backarc rifts and spreading centres bear any detectable contributions from the subducted Pacific Plate in terms of arc-like low Nb/U or Ce/Pb (refs 41 , 43 ). We conclude that neither the Vitiaz arc (pre-Lau Basin opening), nor the current plate tectonic setting has modified or is modifying the supra-subducted Pacific Plate mantle wedge currently serving as a magma source below the northwestern Lau Basin. Although substantial overlap exists, the abundances of the light-middle rare earth elements (REEs) in basalt samples increase from south to north in the northwestern Lau Basin. Strikingly, basalts from the CLSC are among the most depleted in terms of REE among the full spectrum of global MORB [51] , [52] , and have consistently and markedly light δ 57 Fe compared with global MORB, likely related to the refractory nature of the sub-CLSC mantle source [49] . The RR have slightly convex-upward, chondrite-normalized REE abundance patterns, consistent with some degree of partial melting in the presence of residual garnet [41] , [43] . The key question that remains therefore is: ‘do the south-to-north variations in the geochemical characteristics of magmas erupted in the northwestern Lau Basin reflect mantle compositional variations independent of the Samoan Plume, or has ingress of some or all of the Plume components from the latter been superimposed on a prevailing CLSC-type mantle?’ To explain the Hf-Nd-He isotope signals in the northern Lau Basin, we make use of the generally coupled behaviour of the Hf-Nd isotope systems in mantle-derived magmas. We emphasize a number of features of the data in Fig. 2 . Although there is overlap between the three spreading centres and rifts, the northwestern Lau Basin suites become progressively more radiogenic in terms of Hf-Nd isotopic character from the RR through the NWLSC to the CLSC. Variable degrees of partial melting of a single common source cannot explain this diversity, and the strongly radiogenic character of the CLSC ( ε Nd ≤+13) is consistent with a mantle source that has experienced an ancient melt depletion episode(s). A range of mantle sources is required to account for the spread of Hf-Nd isotopic data, adequately explained by mixing between two mantle components. We note further that our data for the RR and the NWLSC suites are well correlated in ε Hf versus ε Nd with a curvature that is deviant from the global MORB-OIB array ( Fig. 2 ). Such curvature can be attributed to mixing between two components with differing Hf/Nd (ref. 53 ) and distinct isotope compositions. Assuming a mantle source mixing process is occurring beneath the Lau Basin, the radiogenic component is plausibly the local depleted wedge-mantle, represented by samples from the CLSC. Progressive decrease in ε Hf versus ε Nd requires mixing between such ‘ambient’ Lau mantle and a less-radiogenic Hf-Nd component (that is, ε Hf ~+7; ε Nd ~+4), consistent with FOZO. Although published data for the northwestern Lau Basin include some samples that are slightly less radiogenic in terms of Hf-Nd isotopic character than FOZO, a critical point is there are none that extend very far towards the strongly unradiogenic, archetypal EM2 end-member represented by the Malu portion of the Samoan islands [13] . We note further that some of the other literature data apply to dredged samples recovered before the era of multi-beam swath mapping and targeting of morphologically young volcanic structures, unlike those of the NoLauVE voyage [47] . It is possible these samples are significantly older than those recovered during NoLauVE [47] , and their compositions may reflect different conditions of magma generation. The comparison in Fig. 3 of our Nd data with 3 He/ 4 He for the same samples and published values for Samoa is instructive. First, a value of 143 Nd/ 144 Nd=+0.51285 ( ε Nd ~4) divides >95% of the samples from the northwestern Lau Basin from Samoa. Only the DV sample has a lower ε Nd at R / R A <10. Second, although considerable scatter at any given 143 Nd/ 144 Nd exists in terms of 3 He/ 4 He, both for the northwestern Lau Basin and Samoa, the majority of the former are encompassed by an envelope of mixing trajectories defined by DMM (CLSC) and FOZO end-members, whereas Samoa fans between DMM, EM2 and FOZO. The mixing lines are a function of absolute abundances of Nd and He, 143 Nd/ 144 Nd and 3 He/ 4 He of the end-members. We note further the high 3 He/ 4 He samples are also characterized by Ne (same aliquots) and Xe (samples from ref. 41 ) isotopic values consistent with a FOZO end-member [1] , [2] , [3] . Jackson et al . [16] present evidence that the high 3 He/ 4 He component in Samoan lavas has other isotopic similarities with a group of OIB suites that occur in the southern hemisphere. These are isotopically distinct from high 3 He/ 4 He OIB in the northern hemisphere, and stimulated the hypothesis of austral (FOZO-A) and boreal (FOZO-B) components in the mantle. Although the Hf-Nd isotopic data for the Lau Basin extend to the FOZO-A component, the mixing envelopes shown in Fig. 3 for current data do not exclude the possibility of FOZO-B involvement. Published Nd-Pb-Sr isotopic data for the Lau Basin in comparison with Samoa are shown in Supplementary Figs 1 and 2 ; the great majority are consistent with mixing between a DMM and FOZO component, and do not extend towards the EM2, HIMU and EM1 components seen in the Samoan data arrays. Decompressional mantle melting during upwelling has previously been proposed to explain OIB-type volcanism in the northern Lau Basin [42] , [54] . OIB components are assumed to have lower solidus temperatures at any given pressure than DMM sources, and preferentially melt but mix with and trigger partial melting of the relatively refractory DMM matrix [42] , [54] . The two-component mixing invoked here to create the trend observed in Fig. 2 requires the specific plume (OIB) end-member has a very narrow Hf-Nd isotope composition, unlike the total range documented for the Samoan Plume [13] , [55] . On the basis of geographic isotopic provinciality in the subaerial and submerged portions of the Samoan chain, Jackson et al . [13] have recently proposed a geometric model for the structure of the Samoan Plume: a sheath of FOZO encloses stringers of DMM, EM2 and HIMU. The location of the EM1 component manifest in mixing arrays with FOZO, characteristic of the ‘rejuvenated’ volcanism on Savai’I, Upolu and Tutuila, remains uncertain. Our primary conclusion from the sum of all the available trace element and isotopic data for the northwestern Lau Basin is that mixing is occurring in the underlying upper mantle between a local DMM component, similar to that sampled at the CLSC and a FOZO component that diminishes in volumetric proportion southward from the RR through the NWLSC towards the CLSC. The most plausible source of the FOZO component is through advection of a portion of the Samoan Plume southwards through the tear in the Pacific Plate. If so, based on primordial Xe isotope signatures for the northern Lau Basin [3] , the FOZO-A component of the Samoan mantle plume is also of primordial origin, despite its Nd isotope excursion from a non-chondritic primitive mantle (FOZO-B). There is no evidence that the other mantle components identified in the Samoan Plume are accompanying the FOZO-A component in the Lau backarc basin. These features are consistent with the model of Jackson et al . [13] , which invokes an external sheath of FOZO hosting stringers of other mantle components, whereby only the southern portion of the external FOZO sheath is advected southwards. Alternatively, it may be the stringers have already been melted out of the rising plume, with only the FOZO fraction remaining to be advected at shallow mantle depths. The slight residual garnet signature in the RR samples suggests some melting of the ingressing plume component is occurring deeper in the northern Lau Basin than to the south. There are nevertheless some difficulties with our general conclusion. For example, Jenner et al . [43] emphasize the high Cu contents of the NWLSC, the markedly low Cu abundances of Samoan lavas and the possibility that three-component mixing between a DMM source (CLSC), a distinctively high-Cu mantle source of the NWLSC and a low-Cu Samoan Plume component is required to account for the abundances of this element in the different spreading centres and rifts of the northwestern Lau Basin. Jenner et al . [43] also note despite the lack of a typical subduction zone signature, marked enrichments of hydrothermally mobile As and Tl in the RR, which points to local magma source complexity. The presence of another mantle plume in the region has also been suggested; for example, the post-subduction alkalic volcanism of Fiji became OIB-like following the initial opening of the Lau Basin [56] . Resolution of a northern (Samoan) versus potential southern (Fijian) source could be resolved with a systematic study of the numerous spreading centres and rifts that lie to the north of Fiji between the North Fiji and Lau basins. Nevertheless, the sum of the available data for the northwestern Lau Basin is most straightforwardly and currently explained by selective ingress of the FOZO component of the Samoan Plume, and variable extents of mixing of this component with an ambient wedge mantle sampled in its purest form along the CLSC. Sample dissolution and purification Twenty-five dredged seafloor samples were analysed for their Hf and Nd isotope compositions. The exact sample powders were used from the RR and NWLSC and a sample from the DV that have previously been analysed for their major and trace elements [43] and their He isotope compositions [2] . Approximately 100 mg of powdered sample material was dissolved in 15 ml Teflon vials in a HNO 3 -HF acid mixture on a hotplate at ~150 °C for 24 h. Afterwards samples were subsequently dried down and repeatedly re-dissolved and dried in concentrated nitric acid with traces of HCl and HF until a clear sample solution was achieved. Both, Hf and Nd were purified from the same dissolution batch, including Fe for subsequent Fe isotope analyses, and sequentially extracted from the rock matrix using a combination of Biorad MX1 resin (for Fe), Eichrom Ln-Spec and Tru-Spec a resin. Details of the chemical procedures are similar to those reported for Hf (ref. 57 ) and for Nd (ref. 58 ). Hafnium and Neodymium isotope analyses Hafnium and Nd isotope ratios were analysed using a Thermo-Fisher Neptune plus multi-collector mass spectrometer with inductively coupled plasma source, housed at the ANU. Hafnium was introduced using a mixture of weak nitric and fluoric acids via a Cetac Aridus II introduction system for dry plasma conditions. Neodymium was introduced with weak nitric acid using a cyclone spray chamber and analysed in wet plasma conditions. All samples were normalized to a JMC-475 Hf standard isotope value of 176 Hf/ 177 Hf=0.282160 and a La Jolla Nd standard isotope value of 143 Nd/ 144 Nd=0.511859 from standard values obtained during the analytical sessions with 176 Hf/ 177 Hf=0.282145±9 (JMC-475) and 143 Nd/ 144 Nd=0.511829±20 (La Jolla), respectively. Blanks for both elements were constantly low during the course of the study with Hf<10 pg and Nd<30 pg. Samples are reported in the epsilon notation, defined as the deviation from the chondritic uniform/unfractionated reservoir times 10,000 using values by ref. 59 . How to cite this article: Nebel, O. and Arculus, R. J. Selective ingress of a Samoan plume component into the northern Lau backarc basin. Nat. Commun. 6:6554 doi: 10.1038/ncomms7554 (2015).